RNA sequencing reveals the complex regulatory network in the maize kernel RNA sequencing can simultaneously identify exonic polymorphisms and quantitate gene expression. Here we report RNA sequencing of developing maize kernels from 368 inbred lines producing 25.8 billion reads and 3.6 million single-nucleotide polymorphisms. Both the MaizeSNP50 BeadChip and the Sequenom MassArray iPLEX platforms confirm a subset of high-quality SNPs. Of these SNPs, we have mapped 931,484 to gene regions with a mean density of 40.3 SNPs per gene. The genome-wide association study identifies 16,408 expression quantitative trait loci. A two-step approach defines 95.1% of the eQTLs to a 10-kb region, and 67.7% of them include a single gene. The establishment of relationships between eQTLs and their targets reveals a large-scale gene regulatory network, which include the regulation of 31 zein and 16 key kernel genes. These results contribute to our understanding of kernel development and to the improvement of maize yield and nutritional quality. Maize is both a model organism for genetic studies and an important crop for food, fuel and feed [1] . Maize kernels accumulate a large amount of storage compounds such as starch, oil and protein. Understanding the genetic regulation of their synthesis and accumulation will be of great value to maize improvement for yield and nutritional quality. In the last decades, many genes that are essential for maize kernel development and nutrient accumulation have been characterized using genetic mutants or map-based cloning methods [2] , [3] . Linkage or association analyses have identified more than a hundred of loci or candidate genes underlying kernel-related traits [4] , [5] . Moreover, the transcriptome profiles of maize kernel have already been analysed in two elite inbred lines [6] , [7] , [8] , identifying candidate genes and coexpression networks involved in kernel developmental pathways. However, our understanding of the processes and the gene regulatory networks in maize kernels remain limited. With the development of technology and significant reduction in the cost of next-generation sequencing, RNA-seq technology has been successfully used for both single-nucleotide polymorphism (SNP) detection and expression quantitative trait loci (eQTL) analysis to reveal gene regulatory networks that are active in specific tissues [9] , [10] . In this study, we explore the gene expression profiles of the developing maize kernel by RNA sequencing of 368 inbred lines at 15 days after pollination (DAP). Our purpose is to explore the sequence diversity across the inbred lines, especially in the gene regions, and to discover the gene regulatory networks employed in immature maize kernels. The results show that there are extensive gene expression variation and sequence diversity among the inbred lines and 931,484 of 1,026,244 high-quality SNPs are mapped to the gene regions. The genome-wide association study (GWAS) identifies 16,408 eQTL; 95.1% of the eQTLs are within a 10-kb region and 67.7% of them include a single gene. The establishment of relationships between eQTLs and their targets reveals a large-scale gene regulatory network. These results can be used to systematically examine the potential effects of gene variants on kernel-associated traits and biological pathways. RNA-seq reveals extensive diversity in maize transcripts The poly(A) + transcriptome of immature kernels (15 DAP) from 368 maize inbred lines were sequenced using 90-bp paired-end Illumina sequencing with libraries of 200-bp insert sizes. After filtering out reads with low sequencing quality, 70.1 million reads were maintained in each sample ( Supplementary Data 1 ). In total, 25.8 billion high-quality reads were obtained. On average, 71.0% of the reads were mapped to the B73 reference genome (AGPv2) and 70.3% of the reads to the maize annotated genes (filtered-gene set, release 5b). Among the genes with RNA-seq reads, 71.6% have coverage of >50% of the gene length ( Fig. 1a ). Of all the reads mapped to the genome, 83.5% were mapped uniquely and these reads were used to build the consensus sequence for each sample ( Supplementary Data 1 ). 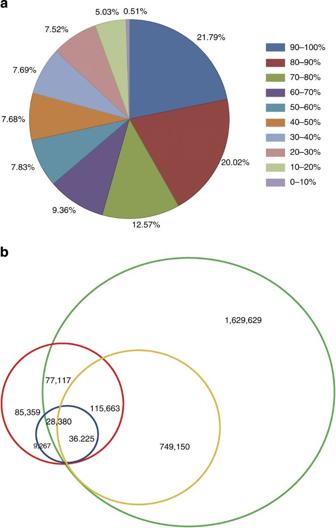Figure 1: Gene coverage by reads and the comparison of SNPs with those from NAM and B73/Mo17. (a) Gene coverage was calculated as the percentage of the gene region covered by reads out of the total gene length. (b) Red circle stands for SNPs of NAM population, blue circle stands for SNPs of B73/Mo17, and green circle and yellow circle stands for SNPs of this study before and after filtering sites with a missing rate >0.6, respectively. After quality control, we identified totally 3,619,762 SNPs using B73 as the reference by a two-step procedure with multiple criteria [11] , [12] ( Table 1 ). Among them, 2,636,164 SNPs were in the exons, which is 5.6 times greater than that previously reported in a group of six elite maize inbred lines (468,900 exonic SNPs) [13] , 7.5 times higher than that reported in the nested association mapping (NAM) population (352,000 exonic SNPs) [14] and 35.7 times higher than that reported between B73 and Mo17 (73,900 exonic SNPs) [14] . Moreover, 69.7% of SNPs in the NAM population and 87.5% of SNPs in the B73/Mo17 were included in our SNP set ( Fig. 1b ). Overall, our SNP data set included 1.6 million of novel SNPs. Compared with the B73 reference genome, the mean number of loci carrying the alternative allele of any given inbred line was 235,651, with a range from 101,020 to 313,630 SNPs ( Supplementary Data 1 ). Figure 1: Gene coverage by reads and the comparison of SNPs with those from NAM and B73/Mo17. ( a ) Gene coverage was calculated as the percentage of the gene region covered by reads out of the total gene length. ( b ) Red circle stands for SNPs of NAM population, blue circle stands for SNPs of B73/Mo17, and green circle and yellow circle stands for SNPs of this study before and after filtering sites with a missing rate >0.6, respectively. Full size image Table 1 Summary of SNPs in 368 maize inbred lines. Full size table Missing genotypes ( Supplementary Table S1 ) were imputed using fastPHASE [15] . By randomly masking ~1% of SNP sites, a simulation was performed to determine the imputation accuracy ( Supplementary Fig. S1 ). The results indicate that the imputation accuracy was 99.3% when the missing data rate cutoff value was set to 0.6. Therefore, 1,026,244 SNPs with a missing data rate of <0.6 were used for imputation to infer missing genotypes. All these SNPs were named according to their chromosome positions in the B73 reference genome (Methods). SNP quality control and distribution To evaluate the reproducibility of genotyping by RNA-seq, we first compared the genotypes of three pairs of biological replicates SK, Han21 and Ye478. The concordant rates between each pair of replicates were >99% ( Supplementary Table S2 ), indicating that our sequencing and SNP calling methods were reproducible. Second, the genotypes of this study were compared with the genotypes determined by the MaizeSNP50 BeadChip [16] . By comparing the overlapping genotypes, the concordant rate between the genotypes determined by RNA-seq and those by the MaizeSNP50 BeadChip was 98.6% before imputation and 96.7% after imputation ( Supplementary Table S3 , Supplementary Fig. S2 and Supplementary Data 2 ). Given the significant difference of the minor allele frequency (MAF) of the overlapped SNPs from that of the non-overlapped SNPs ( Supplementary Fig. S3 ), we further compared the concordant rates of SNPs with different MAFs and found that all the SNPs have concordant rates higher than 96% ( Supplementary Table S4 ). Considering that most of the SNPs in the MaizeSNP50 BeadChip are common, 355 SNP sites containing newly identified rare alleles were randomly selected and validated across 96 inbred lines by the Sequenom MassArray iPLEX genotyping system ( Supplementary Table S5 ). In addition, we amplified ten genes by PCR from genomic DNA and sequenced these PCR products using an ABI3730. The 201 SNPs detected by RNA-seq in these genes had a mean concordant rate of 96.1% with those detected by sequencing PCR products from genomic DNA ( Supplementary Table S6 ). These data indicate that the SNP accuracy in the current study is high and comparable with previous studies in maize [13] , [14] . Among the 1,026,244 SNPs, 931,484 were mapped to the gene regions of 23,106 genes (filtered-gene set, release 5b), accounting for 90.8% of the SNPs ( Supplementary Table S7 ). On average, there are 40.3 SNPs per gene ( Supplementary Data 3 ). The distribution of SNPs in various regions of transcripts was also compared, showing that 3′-untranslated regions have the highest SNP densities (one SNP per 37 bp), followed by the CDS (coding DNA sequence) and 5′-untranslated region (one SNP per 62 bp and one SNP per 61 bp; Supplementary Fig. S4 ). Overall, SNP density in the transcript region is approximately one SNP per 54 bp. Compared with the SNPs in the NAM population, more rare alleles and more genic alleles are identified in this study ( Fig. 2 ). These newly discovered variants showed a similar ratio of transition/transversion rate with known variants ( Supplementary Table S8 ). Of all the SNPs in gene regions, 5,146 SNPs were predicted as large effect variations, including 2,347 SNPs predicted to cause nonsense mutations, 112 SNPs predicted to cause start codon disruption, 571 SNPs predicted to cause stop codon disruption and 2,116 SNPs predicted to destroy splice sites ( Supplementary Data 4 ). In the CDS regions, a total of 244,280 SNPs (48.3%) were annotated as synonymous mutations and 259,465 SNPs (51.3%) as non-synonymous mutations ( Supplementary Table S9 ). 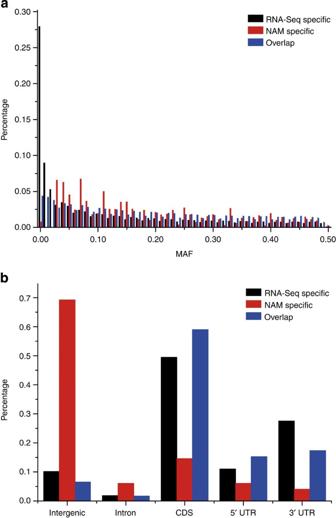Figure 2: Comparison of the newly identified SNPs with the SNPs in NAM. (a) MAF of SNPs. (b) The distribution of SNPs in the genome. Figure 2: Comparison of the newly identified SNPs with the SNPs in NAM. ( a ) MAF of SNPs. ( b ) The distribution of SNPs in the genome. Full size image The distribution of SNPs and genes along the chromosomes was calculated using 1-Mb sliding windows ( Supplementary Fig. S5 ). As expected, the SNP density is related to the gene density. On all chromosomes, the SNP density is low in regions around centromeres, which are also genomic regions with low gene densities; however, exceptions to this correlation could be found, such as regions with high gene density and low SNP density. Because of the sample size and to the inherent relationship between those samples, the overall genome diversity among the 368 inbred lines has a Watterson’s θ of 0.0196, which is much higher than that reported previously [13] , [14] . The gene expression profile is highly variable To quantify the expression of known genes and transcripts, read counts for each whole expressed gene and individual transcripts of the gene were calculated and scaled according to the definition of RPKM (reads per kilobase of exon model per million mapped reads) [17] . The 28,769 genes and 42,211 transcripts having mapped sequencing reads in >50% of the inbred lines were used for eQTL mapping. Of the expressed genes, 97.3% had a mean quantification of more than 10 mapped reads per inbred line, 73.6% had more than 50 reads and 64.1% had more than 100 reads ( Supplementary Fig. S6 ). On average, there are 1,540.7 reads for each whole gene and 1,050.2 reads for each individual transcript. The 100 most highly expressed genes in maize kernel at 15 DAP are listed by the order of mean expression in population ( Supplementary Table S10 ). These genes include members of the globulin, oleosin and zein gene families, as well as other important genes responsible for grain filling. Of the 100 most highly expressed genes, 30 genes were members of the zein gene family, which is in agreement with a previous report on gene expression in maize kernel at 15 DAP [7] . The gene expression profile is highly variable among inbred lines. First, the transcripts of 17,240 genes were detected in all the inbred lines, which may be defined as the core expressed genes of maize kernels at 15 DAP. The remaining 11,529 genes were only detected in some of the inbred lines and absent in other inbred lines. Second, the expression levels of the whole genes and individual transcripts were highly variable across inbred lines ( Table 2 ). Significantly, there are 5,246 genes and 9,233 transcripts that showed a range of expression variation greater than fourfold. Through gene ontology (GO) enrichment analysis [18] , the above 5,246 genes with large expression difference among inbred lines were predicted to be involved in protein metabolism and biosynthetic processes ( Supplementary Fig. S7 ). Table 2 Expression variation for the whole genes and individual transcripts. Full size table Large-scale local and distant eQTLs are discovered by GWAS For the purpose of GWAS analysis, SNPs with a MAF of <5% were filtered out ( Supplementary Fig. S8 ). The resulting 525,105 (51.2%) SNPs were merged with the SNP data from the MaizeSNP50 BeadChip to represent the genotypes of the individual inbred lines; the merged data sets included 558,650 SNPs. Considering the population structure, genetic relatedness among the inbred lines ( Supplementary Fig. S9 ) and the main confounding factors of expression variability, the linear mixed model in the TASSLE software [19] was used for association analysis of the expression levels of 28,769 genes (after normal quantile transformation). The validity of association significance was further examined by including the hidden confounding factors of expression variability in the model, which removed the possible artefacts introduced by confounding factors in gene expression [20] . The quantile–quantile plot resulting from GWAS for 100 randomly selected genes was shown in Supplementary Fig. S10 . This GWAS revealed 591,470 significant associated SNPs by controlling false discovery rate (FDR) of 0.05 with the Benjamini–Hochberg (BH) method (BH rejection threshold: P <2.12 × 10 −6 ). For the 42,211 transcripts, 785,548 significant associated SNPs were detected by controlling FDR at the same level (BH rejection threshold: P <1.89 × 10 −6 ). A two-step method was applied to deal with the association of multiple SNPs with one trait, leading to the identification of eQTL regions ( Supplementary Fig. S11 ). First, we identified 54,764 candidate eQTL from 591,470 significantly associated SNPs by grouping SNPs that are separated by an interval of <5 kb. The most significantly associated SNP in each eQTL region was defined as the lead SNP and the association significance ( P -value) of an eQTL is represented by its lead SNP. Second, the lead SNP of a candidate eQTL was compared with all of the candidate eQTL of the same gene one by one. If the linkage disequilibrium (LD; r 2 ) between this candidate eQTL and another more significant candidate eQTL is >0.1 (a LD decay cutoff value used in diverse maize lines [14] , [21] ), this candidate eQTL will be removed, which substantially avoids the false positives. 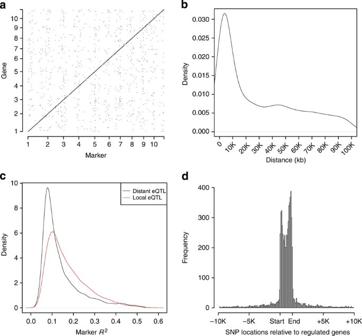Figure 3: GWAS for gene expression. The associations of the SNPs and the expression levels of each gene across 368 maize inbred lines are performed using linear mixed model. (a) The start position of the mapped genes in the maize genome is plotted against the position of the associated SNPs with the Bonferroni threshold (P<3.11 × 10−12). (b) The density of the distances between the lead SNP of each eQTL and its associated genes. If the lead SNP is in the upstream of the target gene, the distance from the SNP to the transcription start site was counted. If the lead SNP is in the downstream of the target gene, the distance from the SNP to the transcription end site was counted. Lead SNPs located in the annotated gene regions were excluded to avoid overweighting from enriched SNPs. (c) The distribution of the effects of local and distant eQTLs. Red line represents local association. (d) The distribution of the lead SNPs in local eQTLs. Finally, 16,408 eQTLs were identified for 14,375 genes ( Table 3 ). Among the genes with eQTLs, 12,605 genes (87.7%) had only 1 eQTL, 1,535 genes had 2 eQTLs and 235 genes had 3 or more eQTLs ( Supplementary Fig. S12 ). In an analogous manner, 22,028 eQTLs were identified for 19,873 transcripts, corresponding to 15,437 genes ( Table 3 and Supplementary Fig. S13 ). Table 3 Summary of eQTLs in developing maize kernel by GWAS. Full size table When the start positions of the mapped genes with eQTLs were plotted against the position of the lead SNP of the eQTL, even after controlling genome-wide error of 0.05 with Bonferroni method (Bonferroni threshold: P <3.11 × 10 −12 ), a strong enrichment was observed along the diagonal, indicating a strong local regulatory relationship of gene expression ( Fig. 3a ). Excluding the eQTLs where the lead SNPs were located within the target gene, the density of lead SNPs peaked around the gene and dropped sharply down to plateau at ~20 kb away from their associated gene ( Fig. 3b ). Therefore, the eQTLs with lead SNPs located within the gene or up to 20 kb from their associated gene were defined as local eQTLs. Otherwise, eQTLs were designated as distant eQTLs. On the basis of this criterion, 9,050 local eQTLs (55.2%) and 7,358 distant eQTLs (44.8%) were detected ( Table 3 ). As local eQTLs tend to have larger effects than distant eQTLs ( Fig. 3c ), the proportion of local eQTLs gradually increased from 55.2 to 68.7% when the P -value was adjusted from the BH threshold to the Bonferroni threshold ( Supplementary Fig. S14 ), which is consistent with previous reports in Arabidopsis and maize [22] , [23] . The resulting eQTLs for individual transcripts showed similar trends in local and distant regulatory patterns, as well as in effect differences ( Supplementary Figs S14 and S15 ). Figure 3: GWAS for gene expression. The associations of the SNPs and the expression levels of each gene across 368 maize inbred lines are performed using linear mixed model. ( a ) The start position of the mapped genes in the maize genome is plotted against the position of the associated SNPs with the Bonferroni threshold ( P <3.11 × 10 −12 ). ( b ) The density of the distances between the lead SNP of each eQTL and its associated genes. If the lead SNP is in the upstream of the target gene, the distance from the SNP to the transcription start site was counted. If the lead SNP is in the downstream of the target gene, the distance from the SNP to the transcription end site was counted. Lead SNPs located in the annotated gene regions were excluded to avoid overweighting from enriched SNPs. ( c ) The distribution of the effects of local and distant eQTLs. Red line represents local association. ( d ) The distribution of the lead SNPs in local eQTLs. Full size image When the distribution of local eQTLs, relative to their target genes, was considered, most lead SNPs of the eQTL were located within the gene region ( Fig. 3d ). Interestingly, local eQTLs had two peaks within exonic regions at the 5′- and 3′-regions, respectively. The location of local eQTLs perhaps indicates that the 5′- and 3′-sequences of complementary DNAs are most important for the regulation of gene expression or the stabilization of mRNA. The eQTL analysis reveals complex regulatory networks After the two-step analysis, eQTL regions were defined by both the lead SNP and significantly associated flanking SNPs. 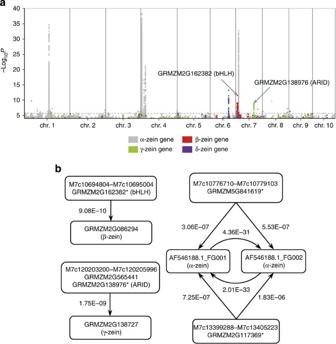Figure 4: The inferred regulatory network of the zein family genes. (a) SignificantP-values from linear mixed models based on the predicted gene expressions of zein family genes. Thexaxis indicates the SNP location along the ten chromosomes; theyaxis is the −log10(P-value, partialF-test) of the association. The TF, which was located in an eQTL and included its lead SNP, is shown along the top of the eQTL region. TheP-values for α-zein, β-zein, γ-zein and δ-zein are indicated by different coloured dots. The boundary of BH threshold (P=2.12 × 10−6) is indicated by a dash line. (b) Directed subnetworks of several zein family genes. eQTLs with candidate regulators are connected to their target genes based on significant associations. The directions of the arrows point from eQTLs to their target genes. The eQTL region is represented by two significantly associated flanking SNPs. The star symbol marks the gene, which contains the lead SNP of its located eQTL. The gene names in italics represent the genes cloned from opaque mutants. Among the 16,408 eQTLs identified by the BH threshold, 15,598 eQTLs were contained within a 10-kb region of the genome, which accounted for 95.1% of all the detected eQTLs ( Table 4 ). By the Bonferroni threshold, the percentage of small-size eQTLs dropped down, but still 93.2% of the eQTL were defined within a 10-kb region. Table 4 The size and average effect of eQTL region from gene expression. Full size table Over 67.7% of eQTL regions (11,115 eQTLs) were found to include only a single gene ( Supplementary Data 5 ) and were involved in the regulation of 10,044 genes. The establishment of gene-to-gene relationship revealed the specific regulatory network affecting maize kernel development, although parts of which may be shared between tissues [24] . In the regulatory networks, 455 transcription factors (TFs) were found to regulate gene expression and 44 of these TFs were predicted to regulate the expression of other TFs ( Supplementary Table S11 ). Interestingly, eQTLs for 16 key genes, which have been reported to show visible mutant phenotypes in maize kernel development [25] , are discovered ( Table 5 ). Among them, 14 genes have one eQTL and 2 genes have two eQTLs. The mn1 gene, which encodes an endosperm-specific cell wall invertase and determines the kernel size [26] , is predicted to be regulated by a gene encoding the UDP-glycosyl transferase ( Supplementary Fig. S16 ). Table 5 Regulation of some key genes important for maize kernel development. Full size table Considering the high-level expression of zein genes in maize kernel at 15 DAP, the expression of 34 zein family genes was further analysed, including 29 α-zeins, 3 γ-zein, 1 β-zein and 1 δ-zein. The 28 α-zeins were predicted to be regulated by at least 1 eQTL. Eight α-zeins were predicted to be regulated by only local eQTLs, 18 α-zeins were predicted to be regulated by 1 or more distant eQTL and 2 α-zeins were predicted to be regulated by both local and distant eQTLs. The δ-zein gene was predicted to be regulated by a local eQTL, with a significant P -value of 6.48 × 10 −14 . The 15-kDa β-zein was regulated by a bHLH TF (GRMZM2G162382) and a 27-kDa γ-zein was regulated by an ARID TF (GRMZM2G138976; Fig. 4a ). By connecting regulators and their target genes, a network involving zein genes and opaque genes were illustrated ( Fig. 4b ). Two eQTLs on chromosome 7 were identified to regulate two α-zein genes, and these two zein genes were also strongly regulated by each other. The regulatory relationships between the β-zein and bHLH gene, as well as the γ-zein and ARID gene were supported by the consistency of their expression patterns during kernel development [8] ( Supplementary Fig. S17 ). Moreover, several binding motifs of bHLH were found in the upstream region of the β-zein gene, indicating a possible direct regulation of β-zein by the bHLH gene. The expression of the above four genes in more than 160 inbred lines were also validated by quantitative reverse-transcription PCR ( Supplementary Table S12 ). Additional coexpression analysis detected three distinct clusters, including a large cluster with all α-zeins ( Supplementary Fig. S18 ). Figure 4: The inferred regulatory network of the zein family genes. ( a ) Significant P -values from linear mixed models based on the predicted gene expressions of zein family genes. The x axis indicates the SNP location along the ten chromosomes; the y axis is the −log 10 ( P -value, partial F -test) of the association. The TF, which was located in an eQTL and included its lead SNP, is shown along the top of the eQTL region. The P -values for α-zein, β-zein, γ-zein and δ-zein are indicated by different coloured dots. The boundary of BH threshold ( P =2.12 × 10 −6 ) is indicated by a dash line. ( b ) Directed subnetworks of several zein family genes. eQTLs with candidate regulators are connected to their target genes based on significant associations. The directions of the arrows point from eQTLs to their target genes. The eQTL region is represented by two significantly associated flanking SNPs. The star symbol marks the gene, which contains the lead SNP of its located eQTL. The gene names in italics represent the genes cloned from opaque mutants. Full size image eQTL mapping is a novel way to identify new variants To further evaluate the mapped eQTL in unravelling candidate genes for interested traits, we use provitamin A–carotenoid concentration as an example. Expression of 20 genes in the carotenoid metabolic pathway were correlated with carotenoid concentration ( P -value<0.05, Student's t -test), of which six genes (including two well-studied genes, lcye1 (ref. 27 ) and crtRB1 (ref. 28 )) were found to have eQTLs in this study, co-located with previously identified QTL for carotenoid-related traits in maize kernel [29] , [30] , [31] ( Table 6 ). After further exploiting the genome-wide gene expression results, in addition to lcye1 , 55 genes were correlated with carotenoid concentration at P -value<10 −8 (| r |>0.3, Student’s t -test) level, of which 19 genes had eQTLs co-located with previously identified QTL. The results implied that at least some of these identified genes could be the candidate genes controlling carotenoid biosynthesis. It also suggested that complex traits could be divided into many simple components at the levels of transcription regulation by genome-wide correlation between the gene expression and targeted traits, and eQTL overlapped with expression-phenotype-associated genes were promising variants for target traits. Table 6 List of genes correlated with Provitamin A cartenoid concentration. Full size table We also analysed the coexpression of potential genes ( Table 6 ) with genes included in eQTLs. Three distinct coexpression clusters were detected with several carotenoid-related genes ( Supplementary Fig. S19 ). Five out of six genes in carotenoid metabolic pathway were classified into the coexpression clusters. Some genes in one coexpression cluster, such as crtRB1 , crtRB3 and GGPPS2 , may be due to the consensus variations of common products in the pathway. In this study, the gene expression profiles in developing kernels and the sequence diversity across 368 maize inbred lines were examined by RNA sequencing. In general, deep RNA sequencing, a reduced genome complexity approach, provides adequate sequence depth for SNP discovery in expressed regions without the requirement to sample the whole plant genome [32] . However, there are also some limitations in detecting variation using RNA-seq compared with genomic resequencing. We have carefully taken them into consideration in the experimental design and data analyses in our study. First, maize inbred lines were used to avoid the bias introduced by allele-specific expression. Alternative splicing, another source of bias, leads to error mapping to reads spanning splice junctions. Two or more such reads with high quality (>20), covering each of continuous exons at least 15 bp, were used to support variation near the splicing site. Through deep RNA-seq, we obtained an average of 70 million reads for each inbred line, which resulted in the recovery of 1.03 million high-quality SNPs in the maize genome. The identified SNPs are of significance to the maize research community, especially in exploring the genetic architecture of quantitative traits in maize using GWAS, as genomic SNPs were often used in previous GWASs in maize, including leaf architecture [33] , leaf metabolites [34] and disease resistance [35] , [36] . Most of the newly identified SNPs were mapped to gene regions with an average of 40.3 SNPs per gene, which substantially complemented the maize SNP polymorphisms discovered by genome resequencing [13] , [14] . There is a high concordance between our SNP data determined by RNA-seq and those by the MaizeSNP50 BeadChip, the Sequenom MassArray iPLEX genotyping system and direct genomic PCR amplicon sequencing ( Supplementary Tables S3–S6 ). Occasional low concordant rate at a few SNP loci and inbred lines may be explained as follows. First, plants tend to have a high frequency of intragenomic duplications and (ancient) polyploidy [37] , highlighting the difficulty in discriminating true SNPs from polymorphisms due to the alignment of paralogous sequences. Second, copy number variation, which is common among maize inbred lines [38] , may also lead to SNP calling errors. Third, insertions and deletions, leading to sequence misalignment, affect SNP calling from RNA-seq data, as shown by the high proportion of SNP sites with low concordant rate near the InDels. Fourth, the maize materials for genotyping by the three platforms are not from the same plants, the residual heterozygosis of inbred lines may also be a factor influencing the concordant rate. Regulation of expression variation may be broadly defined by traditional linkage studies [22] , [39] . In experimental populations from two parental lines, eQTL mapping resolution is limited by population size. In a recent study, the genetic resolution was increased in an association by combining high marker density with diverse Arabidopsis accessions, which accumulated historical recombination and new mutations [40] . The degree of LD in an association panel is a major factor affecting the resolution of QTL mapping. By grouping adjacent associated SNPs using a distance cutoff [40] , [41] , equivalent associations involving markers in local LD can be combined. In inbred organisms, such as Arabidopsis and rice, the resolution of association mapping is limited owing to an overall high LD [42] , [43] . For maize, LD generally decays ( r 2 <0.1) within 2 kb in the founders of NAM population [14] and within 500 bp in our diverse panel ( Supplementary Fig. S20 ), indicating that association studies will generally define QTLs in small regions in such maize populations. However, both population structure and relatedness underlines the complex LD structure between distant markers or even across chromosomes, introducing false-positive associations. This problem can be partially solved by mixed modelling [44] , [45] . Our two-step approach substantially reduced the false positives and allowed us to map many eQTLs into small regions frequently containing a single gene. First, a gene level distant cutoff (<5 kb) was used to group associated SNPs into the gene space as candidate eQTL. In the second step, the LD between the lead SNPs of the candidate eQTL was evaluated, resulting in independent eQTLs ( Supplementary Fig. S11 ). Through this method, 15,598 eQTLs (95.1%) were defined within a 10-kb region and 11,115 eQTLs of them (67.7%) included only a single gene. In conclusion, our two-step approach allows a finer mapping of eQTLs than what can be achieved by simply grouping associated markers with a larger distance cutoff. Although early eQTL studies generally included few lines (<100), this study analysed the expression profiles of 368 diverse maize inbred lines in developing kernel at 15 DAP. The design combining large-scale diversity lines with deep RNA-seq can provide sufficient coverage of gene expression and help to narrow the eQTL to gene level, generating the hypothesis of gene regulatory relationship. The data set in this study has been successfully used in exploring the genetic architecture of oil biosynthesis and accumulation in maize kernel, which is a typical quantitative trait controlled by polygenic loci [46] . The results showed that 74 highly significantly associated loci were responsible for oil concentration and fatty acid composition [5] . Twenty-one of the 74 associated polymorphisms were located in known fatty acid biosynthesis genes, including the three previously reported loci DGAT1-2 , FATB and FAD2 . Here, we analysed the regulatory network of zein genes, which are highly expressed during kernel development at 15 DAP [7] . Among the 34 zein genes detected, 31 were predicted to be regulated by at least one eQTL. The finding of eQTLs for 16 key genes in maize kernel development will help us in the understanding of the regulation of these important genes. By combing the carotenoid phenotype and expression genes in kernel, we identified 19 genes highly associated with the phenotype and located in the known QTL region, including two well studied genes [27] , [28] , which provided good candidates for follow-up studies to explore the genetic basis of carotenoid biosynthesis. These results provide the maize community with a good resource for gene mining and the strategy can also be applied in other kernel-related traits. According to our knowledge, this is the first large-scale unravelling of the regulatory network in maize developing kernel by RNA sequencing, although further experiments will be needed for the confirmation of these regulatory relationships. Plant germplasm and sequencing A maize association mapping panel consists of 508 inbred lines, including tropical, subtropical and temperate germplasms [47] . All 508 lines were divided into two groups (temperate and tropical/subtropical) based on their pedigree information and planted in one-row plots in an incompletely randomized block design within the group with two replicates in Jingzhou, Hubei province of China in 2010. Six to eight ears in each block were self-pollinated, and five immature seeds from three to four ears in each block were collected at 15 DAP. The collected immature seeds in two replications were bulked for total RNA extraction. In total, immature seeds after 15 DAP were collected from 368 maize inbred lines. Total RNA was extracted using Bioteke RNA extraction kit (Bioteke, Beijing, China) according to its protocol. In addition, immature seeds at 15 DAP were also collected from maize inbred line, SK, in the Agronomy Farm, China Agricultural University, Beijing in 2010. Library construction and Illumina sequencing were performed as described in Supplementary Methods . The RNA sequencing was performed twice for SK as a positive control. Reads mapping and SNP calling After removing reads with low sequencing quality and reads with sequencing adapter, Short Oligonucleotide Alignment Program 2 (ref. 12 ) was used to map the paired-end reads against the B73 AGPv2. Only reads that mapped uniquely to the genome were retained for further variation calling. Alignment results were then sorted according to their alignment position on the chromosome and converted to SAM format. Using the Pileup command provided by SAMtools package [11] , consensus sequence was generated with the model implemented in MAQ [48] . Next, we used a two-step procedure to detect SNPs by carefully considering the characteristics of RNA-seq data. In the first step, we identified the polymorphism loci from our population. A population SNP-calling algorithm realSFS, which takes a Bayesian approach [49] , was used to calculate the likelihood of variation for each covered nucleotide from the combined data of all the 368 inbred lines. The variations with probability <0.99 or total depth <50 × were filtered out. To further exclude possible false polymorphic sites caused by intrinsic mapping errors, of which paralogues on the reference genome and mapping bias inherent to the mapping algorithm represent the major sources, we constructed a mapping error set (MES) as follows: read sequences were simulated based on whole maize transcriptome using MAQ, no mutation was generated on those reads sequences (−r 0). We simulated 30 × coverage of the reference genome, that is, ~680 Mb reads. Simulated reads were then aligned to the reference genome and SNPs were identified using the same strategies as in the second step. As we did not generate any mutation while simulation, the resulting SNPs can only explained by false positive caused by incorrectly reads mapping. Those SNPs were termed MES and represent an inherently error-prone set of sites that are incorrectly called owing to the nature of mapping and calling algorithms. Any SNPs that matched the MES were removed. In the second step, we extracted consensus base, reference base, consensus quality, SNP quality and sequencing depth of each polymorphism locus for each inbred line using the Pileup, and then considered the consensus base as the individual genotype with the following requirements: if the consensus base was different from the reference base, the non-reference allele must be the same as the non-reference allele detected from the population and the SNP quality must be ≥20. If the consensus base was the same as the reference base, the consensus quality must be equal to or >20 and the minimal depth must be equal to or >5 × . For sites failed to pass these criterions, we regarded the consensus genotype as unreliable and assigned the individual genotype of those sites as missing. Imputation To infer missing genotypes, we used fastPHASE (version 1.3) [15] , a haplotype clustering algorithm, to impute the missing calls in the genotyping data. fastPHASE is based on the fact that haplotypes in a population tend to cluster into groups over short regions. For our analysis, members of a cluster were allowed to continuously change along the chromosome, according to a hidden Markov model that was applied to impute the missing genotypes. All heterozygous genotypes were masked as missing data. To determine whether the imputation accuracy was affected by the degree of the missing genotyping data, we randomly selected 1% of the SNP sites that with missing rates varied from 10 to 90%. Next, we computed the imputation accuracy for this subset of the SNP sites (368 samples for each site), through randomly masking the genotype of one of the samples with a known genotype. The accuracy of the imputation was measured by the proportion of correctly inferred genotypes of the total masked genotypes. By varying the cutoff rate of the missing data, the imputation accuracy and the total SNP number were compared. Lower missing data cutoff rates had similar accuracy, but more SNP sites were discarded. After imputation, all the SNPs were named according to their physical positions in the B73 AGPv2. The name includes two letters and two numbers, such as M1c379868. The first letter ‘M’ represents maize, the second letter ‘c’ represents chromosome, the number between the two letters represents the chromosome number and the number after the second letter represents the SNP position in the reference genome. Positive control In addition, three inbred lines, each of which consists of two replicates, were added as positive controls to the 368 inbred lines, and the same pipeline with the same parameters was used to perform the SNP calling and imputation. We calculated the concordant rate of each pair of positive control samples before and after imputation. To calculate the concordant rate before imputation, missing genotypes from either positive control sample of the pair were not taken into account. The concordant rate was calculated as the proportion of the genotype that was concordant of the total number of comparable SNP sites. SNP validation By comparing the overlapping SNP set from the same inbred line, we estimated the concordant rate of genotypes called from this study and the Illumina MaizeSNP50 BeadChip. The SNP density of MaizeSNP50 BeadChip (containing 56,100 SNPs) is currently the highest among maize commercial SNP arrays, which are designed from maize genomic SNP, most of the SNPs are common variants. In addition, around one out of three of the SNPs located in gene coding regions. The Illumina SNP data were first mapped to unique positions in the B73 AGPv2 using an in silico mapping procedure, and the genotypes were converted to be relative to the plus strand of the reference genome. The concordant rate was calculated as the fraction of the genotypes that agreed from the total number of overlapping SNPs. In addition, the ‘homozygous concordant rate’ was calculated as the fraction of genotypes that agreed from the total number of overlapping genotypes, which were all homozygous in both data sets. Missing genotypes from either data set were not included in the concordant rate calculation. In addition to overall concordant rates, concordant rates were also calculated for each inbred line and each comparable SNP site. To further validate the SNP containing rare allele, we randomly selected 355 SNPs (MAFu5%) and validated the genotypes in 96 selected maize inbred lines through the Sequenom MassArray iPLEX genotyping system. The concordant rate of genotypes with different classes called from this study and the Sequenom MassArray iPLEX genotyping system was estimated using the same comparing procedure as described in the comparison between the SNP genotypes from RNA-seq and the Illumina MaizeSNP50 BeadChip. SNP annotation SNPs were categorized according to their position (intergenic, intronic, exonic and so on) in the annotated maize genes and maize transcripts (filtered-gene set, release 5b). For multiple transcripts from the same gene, we defined the primary transcript with the longest CDS as the representative transcript, such that one SNP had a definite, unique allocation. SNPs located in the exonic region were further categorized as CDS, 5′- and 3′-region, then normalized by the total length of corresponding regions. For transcripts with more than three exons, we also calculated the number of SNPs from the first exon, the last exon and the middle exons. Depending on whether SNPs caused changes in the coding of an amino acid, SNPs in the CDS region of protein-coding genes were annotated as synonymous or non-synonymous mutations. SNPs that introduced premature stop codons and SNPs that disrupt stop codons, initiation codon or splice site were annotated as large-effect SNPs. The genotype variations between our population and the B73 genome were represented as the substitution type. Overlap with SNPs of previous studies The SNP data of the NAM population were downloaded from the database Panzea [50] . We only compared the SNPs from the exon regions, according to the filtered-gene set (release 5b). We also extracted the SNPs between B73 and Mo17, and compared these SNPs with our data set. LD decay LD ( r 2 ) was calculated for all pairs of SNPs within 250 kb using Haploview [51] . The parameters were set as follows: -n -maxdistance 250 -minMAF 0.005 -hwcutoff 0 -dprime. Average r 2 within a 100-bp sliding window with step length of 50 bp was calculated, and the average pairwise distance was determined to be the midpoint of the window. LD decay curves were then plotted with R script, drawing average r 2 against the marker distance. Quantification of known genes and transcripts To quantify the gene and transcript expression, reads were mapped to all the maize genes (filtered-gene set, release 5b). To determine the read counts of a given gene, we summed reads that uniquely mapped to one transcript of the gene, as well as reads that matched to more than one genomic location in the same or in different transcripts of the gene. As reads are generally shorter than the transcript, a single read may map to multiple isoforms of a gene; therefore, there is some uncertainty when we count the transcript reads. To address this uncertainty, we used the program RSEM [52] , which implements generative statistical models and associated inference methods by estimating maximum likelihood (ML) expression levels using an expectation-maximization (EM) algorithm, to allocate reads that mapped to different isoforms of a gene to a specific transcript. Using RPKM [17] , gene read counts and transcript read counts were then normalized by scaling read counts to a total of one million mapped reads per sample and a total gene and transcript length of 1 kb each. Normal quantile transformation For each sample, we included all genes with a median expression level >0 for analyses after RPKM normalization. One of the assumptions of detecting eQTLs through linear mixed model is that the expression values follow a normal distribution in each genotype classes, which is violated by outliers or non-normality in gene expression estimated from the sequencing reads. The approach to examine the robustness of each individual model is not feasible for the millions of models [53] . Thus, the expression values of each gene were normalized using a normal quantile transformation (qqnorm function in R) [54] . This quantile transformation does not fully solve the problem; it only ensures that the phenotype is normal overall but not necessarily normal within each genotype class. However, with the small effect sizes typical in genetic association studies, quantile transformation is a simple, sensible way to guard against strong departures from modelling assumptions. In an analogous manner, the distribution of expression levels for each transcript is also normalized. Population structure and association analysis To estimate population structure and kinship coefficients, 16,338 SNPs with <20% missing data and MAF >5% were used. STRUCTURE, a Bayesian Markov Chain Monte Carlo (MCMC) programme [55] , was used to infer population structure. Burn-in and MCMC replications were both set at 10,000. The admixture model was used assuming correlated allele frequencies among groups. Five runs at k =3 were performed on the panel, previously divided into three subgroups using 884 SNPs [47] . The results of the replicate runs were integrated using the CLUMPP software [56] . The kinship matrix was calculated with the same 16,338 SNPs using the method of Loiselle et al . [57] The neighbour-joining tree of 368 inbred lines was reconstructed using TreeBeST [58] and the bootstrap support for nodes was estimated to be 100. The trees were visualized using MEGA [59] . To perform PCA on the individual inbred lines, SNPs after imputation were used based on the method from Patterson et al . [60] The first two principal components were used to visualize the genetic relatedness among individuals and investigated groups. Normal quantile transformation was used separately for the expression levels of each gene or transcript. The associations between the extracted SNPs with MAF≥5% and transformed expression traits were performed using a linear mixed model [44] , [45] , incorporating population structure and kinship using TASSEL [19] . The association significance of each SNP was tested using a partial F -test calculated by residual sum of squares (RSS) of full model and reduced model (no marker). We further estimated hidden confounding factors contributing expression variability by Bayesian factor analysis (implemented in PEER [61] ). In addition to population structure, six and eight hidden factors accounting for gene and transcript expression variability were, respectively, retained after training (determined by automatic relevance determination [62] ), which were additionally included in the mixed model to examine the validity of association significance. Heterozygous genotypes called by RNA-seq procedure were excluded in the additional analysis. Multiple testing correction Each of 558,650 SNPs was tested for association with quantification of the 28,769 genes and 42,211 transcripts. To deal with multiple testing problem, this analysis produced a Bonferroni threshold by controlling genome-wide error at level α =0.05 using Bonferroni method ( P <3.11 × 10 −12 or 2.12 × 10 −12 ), which is likely to be conservative given the LD structure across the genome. The BH method was applied to control FDR at level α =0.05. As the BH method is simple to implement and is valid for positively correlated tests, it should be applicable to control for errors even with linked marker QTL tests and should provide a better balance for declaring an excess of false-positive QTLs, sacrificing power to detect QTLs that have smaller effects [63] . Identification of eQTL First, we grouped all the associated SNPs (BH threshold) into one cluster if the distance between two consecutive SNPs is <5 kb. Given previous observations that multiple SNPs within a gene are typically associated with a trait [64] , the clusters with at least three significant SNPs were considered as candidate eQTLs represented by their lead SNP. Second, a candidate eQTL in LD ( r 2 >0.1) with other more significant candidate eQTLs for the same expression trait was regarded as false-positive associations introduced by the LD structure and were then removed. If the significance of two candidate eQTLs is identical, the joint effect of associated SNPs in each eQTL was estimated through multiple linear regression (MLR), using the lm function in the R statistical computing environment. Before fitting the model, each marker was recoded, substituting the value 1 for inbred lines with a given allele and value 0 for all other inbred lines. The model was then fitted using least square estimation. The forward–backward (stepwise) selection of markers on the basis of Akaike information criterion (AIC) was started from fitting the null model (no marker). At each forward step, the global significance of the model was evaluated, as well as the significance of the newly added marker. At each backward step, the least significant marker was dropped from the model. R 2 was calculated as the proportion of total phenotypic variation explained by the optimal regression model. The eQTLs with larger joint effects remained. The degree of LD between two candidate eQTLs was calculated between the lead SNP in less significant eQTLs and the more significant eSNPs in another eQTL. The eQTL was considered local if the lead SNP was found within 20 kb of transcription start site or transcription end site of the target gene; otherwise, the eQTL was considered distant. Given population structure and random genetic background, the effect of each eQTL was estimated by solving linear mixed model [45] . Although non-genetic factors are likely to be important to determine gene expression [65] , the simplicity of this methodology can still be used to unravel the genetic model for gene expression. The expression atlas of maize B73 provided orthogonal information (non-genetic variation) to support the gene regulation via natural genetic variation [8] . Network analysis The genes and their regulators were used to construct a genetic network. One gene that was physically located in an eQTL region and contained the lead SNP of that eQTL was assigned as the regulator. On the basis of a pairwise regulatory relationship, the nodes (genes) were connected by generating a directed edge from the regulator to target gene. The annotation of TFs followed the ProFITS database for maize [66] . GO enrichment analysis GO terms was determined by the web toolkit agriGO [18] and used to assess the biological functionality of a group of genes. When five or more mapped genes were grouped into each GO term, hypergeometric distributions were applied to test the significance against background under the maize genome (filtered-gene set, release 5b). The P -values were adjusted for multiple testing by controlling FDR with the BH method. Carotenoid quantification The 508 inbred lines were divided into two groups (temperate and tropical/subtropical) based on pedigree information and were planted in one-row plots in a completely randomized block design within the group with one replication in Ya’an, Sichuan, China, in 2009. More than 6 plants in each row were self-pollinated and 50 kernels from equally bulked kernels for each line were grounded for carotenoid quantification usingHPLC. Carotenoids, including α-carotene, lutein, β-carotene, β-cryptoxanthin and zeaxanthin, were quantified by standard regression against external standards [67] . The concentration of derived provitamin A (Va) was calculated by the sum of α-carotene, β-carotene and β-cryptoxanthin: Provitamin A=β-carotene+(α-carotene+β-cryptoxanthin)/2. Accession codes: The sequencing data for this project have been deposited in the NCBI Sequence Read Archive under accession code SRP026161 . How to cite this article: Fu, J. et al . RNA sequencing reveals the complex regulatory network in the maize kernel. Nat. Commun. 4:2832 doi: 10.1038/ncomms3832 (2013).